Inhibition of return in the archer fish Inhibition of return is the inhibitory tagging of recently attended locations or objects. It was previously suggested that inhibition of return is a foraging facilitator in visual search. Inhibition of return was first discovered in humans and was demonstrated also in monkeys, yet it has never been demonstrated in non-primates. Here we report the presence of inhibition of return in the archer fish, which shoots down prey on overhanging vegetation, using squirts of water spouted from its mouth. Moreover, we find similar attentional effects for fish as for human participants. Our results show that the generation of inhibition of return does not require a fully developed cortex and strengthen the view that inhibition of return functions as a foraging facilitator. A prominent task used since the 1980's to measure orienting of attention in humans is Posner's cuing task [1] . In this task, a non-predictive peripheral cue (for example, a flickering square) is presented before a target and participants are asked to respond to the appearance of the target (for example, an asterisk). Reaction time (RT) to the target is faster to valid trials (that is, target and cue appear at the same location) than invalid trials (that is, target and cue appear at different locations), at short stimulus onset asynchrony (SOA; the duration from cue appearance until target appearance). For longer SOAs this facilitation effect is reversed, that is, RT is faster for invalid trials than for valid trials. This typical pattern of results for the longer SOAs is known as inhibition of return (IOR). IOR was suggested to promote efficiency of visual search during foraging and scanning the environment for vital information [2] . To scan our environment efficiently, it is preferable not to go back to previously scanned locations, but to move to new areas in the field. It was proposed that IOR is an attentional effect designed to promote just that [2] , [3] . IOR was demonstrated in newborns [4] , [5] and was suggested to be generated by the superior colliculus [6] , [7] , [8] , [9] , [10] . The superior colliculus is a subcortical structure that is known to be involved in programming and execution of eye movements. Additional works have suggested that higher brain regions are also involved in IOR. Dorris et al. [11] used single-unit recordings and electrically evoked saccades to examine superior colliculus involvement in IOR. They concluded that the superior colliculus is not the site of the inhibition, and that it receives downstream input that reduces its responsiveness to visual signals. Although it has been demonstrated that information is remapped in the superior colliculus after saccades [12] , the involvement of parietal areas [13] , and specifically the right intraparietal sulcus [14] , may be required for the maintenance of IOR at cued locations after eye movements. Sereno et al. [15] have recently suggested that reflexive attentional effects, that is, facilitation and IOR, may result from simple neuronal repetition suppression and are actually a property of many brain regions (for a similar suggestion see also Dukewich [16] ). If IOR indeed promotes visual search efficiency and is generated by lower-level regions such as the superior colliculus, which corresponds to the optic tectum in many species, one would expect to find IOR in a wide-spread manner across the animal kingdom. Indeed, IOR was demonstrated in monkeys [17] . However, as far as we know, IOR was never presented in non-primates [18] . The literature on foraging in non-primates suggests that optimal foraging is dependent on the ability to avoid returning to already scanned locations. For instance, it was suggested that bees use different strategies, such as bottom-to-top movement along vertical inflorescences [19] , [20] , foraging along a fixed route (traplining) [21] , scent marking of visited flowers [22] , [23] , [24] and numerical abilities [25] , to avoid returning to already visited nectars and pollens in flowers. In vertebrates, the foraging pattern of the albatross exhibits a power law distribution of flight time intervals [26] , that is, it performs many short flights in limited spatial locations and a small number of long flights between distant locations. Although it was demonstrated that the Drosophila melanogaster fly’s brain inhibits unattended objects while facilitating attended ones [27] , the involvement of attentional processes in optimal foraging has not been considered. Most research has focused on foraging strategies that are specific to the examined species. We suggest that some general attentional processes, such as automatic inhibitory tagging of recently visited places, can be a basic mechanism that facilitates optimal foraging in many species. In fact, inhibitory tagging might be the precursor of other optimal foraging behaviours. Fish have an optic tectum but lack fully developed cortical structures. Hence, we explored whether fish exhibit IOR. We trained three archer fish to perform Posner’s exogenous cuing task [1] ( Fig. 1 ). Our main goal was to examine whether these fish demonstrate the typical shift from facilitation to IOR observed in human participants. We selected this fish species to serve as our model because of its remarkable ability to shoot down insects found on foliage above the water level, and its ability to learn to distinguish between artificial targets presented on a computer monitor in an experimental setting [28] , [29] . Thus, the archer fish can provide the fish equivalent of a monkey or a human subject that can report psychophysical decisions, and make controlled and complex experimental procedures possible. The archer fish in our study have presented similar attentional effects to human participants, demonstrating the presence of IOR even in a spacy lacking a fully developed cortex. 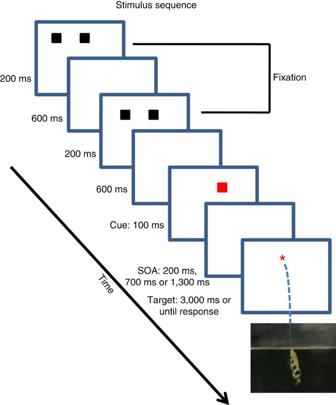Figure 1: The sequence of events in a typical experimental trial. Each trial began with a flickering of two black fixation boxes in one of the four different quadrants on a screen (note that fixation flashed three times, for the sake of demonstration we depicted it only twice). Six hundred milliseconds after fixation disappeared, a red cue box appeared for 100 ms at the left or right fixated location. After a variable SOA of 200 ms, 700 ms or 1,300 ms, a red target asterisk appeared for 3,000 ms or until a response was detected. The target could appear at the cued location (valid trial) or at the opposite location (invalid trial). Figure 1: The sequence of events in a typical experimental trial. Each trial began with a flickering of two black fixation boxes in one of the four different quadrants on a screen (note that fixation flashed three times, for the sake of demonstration we depicted it only twice). Six hundred milliseconds after fixation disappeared, a red cue box appeared for 100 ms at the left or right fixated location. After a variable SOA of 200 ms, 700 ms or 1,300 ms, a red target asterisk appeared for 3,000 ms or until a response was detected. The target could appear at the cued location (valid trial) or at the opposite location (invalid trial). Full size image Archer fish attentional abilities During our experiments, the three fish were trained separately. Each fish swam freely in a water tank. A computer monitor was placed on a glass shelf above water level. The fish were trained to shoot at a target that appeared on the monitor and their movements were recorded through a video camera that was later used to extract RT. After every successful shot, the fish were rewarded with a food pellet. The cue was not predictive regarding target location, that is, the target appeared with the same probability in either the cued or uncued locations. Each trial began with the flickering of two black fixation boxes, presented twice for 200 ms with a 600-ms interval between presentations ( Fig. 1 ). The fixation boxes could appear in one of the four different locations on the screen (see Methods). Six hundred milliseconds after the fixation disappeared, a red cue box appeared for 100 ms at the left or right box position of the fixated location. After a variable SOA (200 ms, 700 ms or 1,300 ms) a red target asterisk appeared for 3,000 ms or until a response was detected. The target could appear at the cued location or at the opposite location. After the target disappeared, a blank screen interval was presented between trials for 10 s. We examined RT of three fish as a function of SOA and validity of the cue ( Fig. 2 ). To detect facilitation and IOR for the different conditions, we conducted an analysis of variance for each fish separately (see Methods). We found that both facilitation and IOR were observed for the archer fish. Fish 1, for example, exhibited facilitation at the first SOA (200 ms) and IOR at the third SOA (1,300 ms), while fish 2 and 3 exhibited facilitation at the second SOA (600 ms) and IOR at the third SOA (1,300 ms). 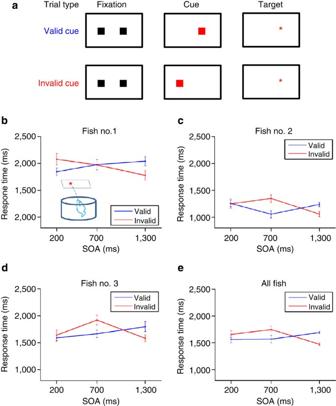Figure 2: Reaction time as a function of SOA and validity for the three fish. All fish completed 14 sessions of the experiment. They all demonstrated facilitation at earlier SOAs, which reversed into IOR at the last SOA. In an analysis of variance a significant interaction between SOA and validity was observed for all the fish (F(2, 26)=5.3,P<0.05;F(2, 26)=6.9,P<0.01;F(2, 26)=6.1,P<0.01, for fish 1, 2 and 3, respectively). This interaction indicated the appearance of facilitation at an early SOA (the first SOA for fish 1,F(1, 13)=5.3,P<0.05, and the second SOA for fish 2 and 3,F(1, 13)=9.9,P<0.01;F(1, 13)=5.5,P<0.05, respectively) and IOR at the third SOA (F(1, 13)=4.9,P<0.05;F(1, 13)=7.4,P<0.05;F(1, 13)=4.9,P<0.05, for fish 1, 2 and 3, respectively). (a) The different experimental conditions. (b–d) The averaged pattern of results for fish 1, 2 and 3 respectively. (e) The averaged pattern of results across fish. The fish successfully responded in 230, 274 and 249 experimental trials (for fish 1, 2 and 3, respectively). Error bars represent one s.e. from the mean using a method to compute the error bars in within-subjects designs33. Figure 2: Reaction time as a function of SOA and validity for the three fish. All fish completed 14 sessions of the experiment. They all demonstrated facilitation at earlier SOAs, which reversed into IOR at the last SOA. In an analysis of variance a significant interaction between SOA and validity was observed for all the fish ( F (2, 26)=5.3, P <0.05; F (2, 26)=6.9, P <0.01; F (2, 26)=6.1, P <0.01, for fish 1, 2 and 3, respectively). This interaction indicated the appearance of facilitation at an early SOA (the first SOA for fish 1, F (1, 13)=5.3, P <0.05, and the second SOA for fish 2 and 3, F (1, 13)=9.9, P <0.01; F (1, 13)=5.5, P <0.05, respectively) and IOR at the third SOA ( F (1, 13)=4.9, P <0.05; F (1, 13)=7.4, P <0.05; F (1, 13)=4.9, P <0.05, for fish 1, 2 and 3, respectively). ( a ) The different experimental conditions. ( b – d ) The averaged pattern of results for fish 1, 2 and 3 respectively. ( e ) The averaged pattern of results across fish. The fish successfully responded in 230, 274 and 249 experimental trials (for fish 1, 2 and 3, respectively). Error bars represent one s.e. from the mean using a method to compute the error bars in within-subjects designs [33] . Full size image To follow the standard analysis procedure used in conventional attention experiments, we also conducted a group analysis for the three fish. Across fish a significant facilitation was observed at the first two SOAs and a significant IOR was observed at the last SOA ( P <0.05 for both comparisons). This observation substantiates our analysis on the single-subject level and demonstrates that facilitation and IOR are present in vertebrates, which are evolutionarily distant from humans. Humans’ attentional abilities The task used in the archer fish experiments is slightly different from the common task used for humans. Commonly, cues and targets are presented at the centre of the screen, whereas here there were four possible locations. To ensure that humans also exhibit IOR in this slightly modified setting, we conducted the same experiment with human subjects. We found that both facilitation and IOR were observed for human participants ( Fig. 3 ). IOR was observed at the 700 ms SOA and was absent at the last SOA (1,300 ms). All archer fish demonstrated IOR at the last SOA. This indicates that although both species demonstrate facilitation at early SOAs and then IOR, the shift to IOR appears earlier for humans. 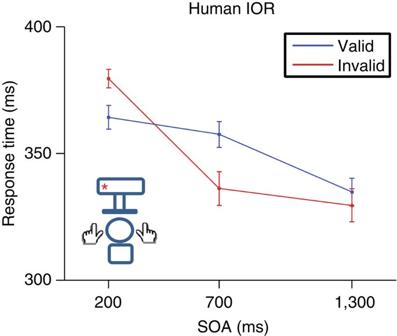Figure 3: Reaction time as a function of SOA and validity for the human participants. As can been seen, human participants demonstrated facilitation at the first SOA, which reversed into IOR at the second SOA. In an analysis of variance, we found a main effect of SOA (F(2, 18)=17.5,P<0.001), which indicated a linear decrease in reaction time as SOA became longer (F(1, 9)=58,P<0.001). Similar to the fish, the interaction between SOA and validity was also significant (F(2, 18)=10.1,P<0.01). This interaction indicated the appearance of facilitation at the first SOA (F(1, 9)=6.4,P<0.05) and IOR at the second SOA (F(1, 9)=9,P<0.05). Each participant completed 96 experimental trials. Error bars represent one s.e. from the mean using a method to compute the error bars in within-subjects designs33. Figure 3: Reaction time as a function of SOA and validity for the human participants. As can been seen, human participants demonstrated facilitation at the first SOA, which reversed into IOR at the second SOA. In an analysis of variance, we found a main effect of SOA ( F (2, 18)=17.5, P <0.001), which indicated a linear decrease in reaction time as SOA became longer ( F (1, 9)=58, P <0.001). Similar to the fish, the interaction between SOA and validity was also significant ( F (2, 18)=10.1, P <0.01). This interaction indicated the appearance of facilitation at the first SOA ( F (1, 9)=6.4, P <0.05) and IOR at the second SOA ( F (1, 9)=9, P <0.05). Each participant completed 96 experimental trials. Error bars represent one s.e. from the mean using a method to compute the error bars in within-subjects designs [33] . Full size image What is the variability across fish and can we compare it to humans? In humans, attentional effects are very robust phenomena at the group mean level, yet much variability in those effects was demonstrated at the individual level [30] . So, it is not surprising to observe differences in the time course of the attentional effects in fish. This was observed in the earlier presentation of facilitation for fish 1 compared with fish 2 and 3 ( Fig. 2 ). Moreover, as can be seen in Fig. 4 , the between-fish variability resembles that of humans in the task used in the present work. 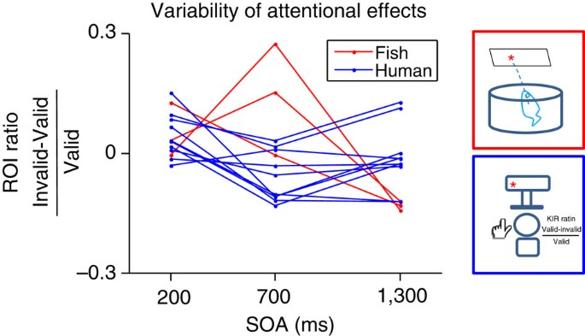Figure 4: Both fish and humans show large variability in attentional effects. IOR as a ratio between the validity effect and RT of the valid condition for humans (blue bars) and fish (red bars). As can be seen, both humans and fish demonstrated some variability in the attentional effect. There is also a difference in the time course of facilitation and IOR between humans and fish. Humans mostly demonstrate facilitation at the first SOA and IOR at the second, whereas fish mostly demonstrate facilitation at the second SOA and IOR at the third. Figure 4: Both fish and humans show large variability in attentional effects. IOR as a ratio between the validity effect and RT of the valid condition for humans (blue bars) and fish (red bars). As can be seen, both humans and fish demonstrated some variability in the attentional effect. There is also a difference in the time course of facilitation and IOR between humans and fish. Humans mostly demonstrate facilitation at the first SOA and IOR at the second, whereas fish mostly demonstrate facilitation at the second SOA and IOR at the third. Full size image This work is the first to demonstrate the appearance of IOR in a non-primate species. We explored the attentional ability of three archer fish using Posner’s cuing task [1] . We found that the fish, similar to humans, demonstrated an early facilitation effect that was superseded by IOR. As previously demonstrated for humans [30] , we found a between-fish variability in the attentional effect. The present work strengthens the role of IOR as a foraging facilitator that inhibits the return to previously attended locations and facilitates the search of new areas in the field [2] , [3] . This view implies that IOR is generated by the superior colliculus [6] , [7] , [8] , [9] , [10] and was present early on in evolutionary development. According to this view, IOR should be found in a wide-spread manner across the animal kingdom and might have implications for the research of non-primate foraging processes. It should be noted that a previous study failed to find IOR in pigeons [18] . As acknowledged by the authors, in that work the pigeons were required to respond to the cue before target presentation. This might have made the cue a rewarding stimulus, and could have enhanced facilitation of the cued location. In the present study, IOR was measured in a similar task to that used for humans (for example, no response to the cue was required). It is widely accepted that attentional orienting in humans involves a frontoparietal network [13] , [31] , [32] . Most of the research on attention has examined humans and monkeys, somewhat neglecting non-primate species. Our work demonstrates that human-like attentional effects, both facilitation and IOR, are observed in the archer fish, which does not have fully developed cortical tissue. Our findings strengthen the view of IOR as a foraging facilitator in visual search that is generated by subcortical brain structures and does not require the involvement of higher cortical regions. The present work demonstrates that in the archer fish such subcortical structures are not only essential, but are sufficient for IOR presentation. In our task the archer fish swam freely during the task, which implies that in order for the cued location to be inhibited, the inhibitory tagging had to be remapped after every movement of the fish. The fact that we still observed IOR at the cued location might indicate that, in contrast to previous suggestions [13] , [14] , a developed parietal cortex is not necessary for remapping the inhibitory tagging provided by the superior colliculus. Behavioural experiment with archer fish All experiments were conducted in accordance with Ben-Gurion University of the Negev regulations and the State of Israel’s laws on animal care and experimentation. Each fish was swimming freely in its tank during the task. A 17-inch computer monitor (DELL, E176FP) was placed on a glass shelf 34.5 cm above water level. The fish were trained to shoot at the target stimuli and were recorded through a 60-Hz video camera (Point Grey, FL2). RT was calculated by measuring the time from target appearance until the fish shot exited the water. After every successful shot, the fish received a pellet of food and the water was cleaned from the glass shelf by the experimenter. The cue was not predictive regarding target location, that is, the target appeared with the same probability in either the cued or uncued locations. In each session each fish was presented with 24 trials, composed of three different SOAs (200 ms, 700 ms or 1,300 ms) and two validity conditions (valid, invalid). The fish were trained on the task until they achieved proficiency before we started to collect data. Each trial began with the flickering of two black fixation boxes (6.6° each side), whose centres were 8.6° from each other. Flickering was achieved by flashing the two fixation boxes three times (that is, they appeared for 200 ms with a 600-ms interval between appearances). The fixation boxes could appear in one of four different locations on the screen, centred 11.5° to the right or left and 15.5° above or below the center of the screen. The cue and target could appear only at the fixated locations (that is, either the right or left box position of the fixation). Six hundred milliseconds after fixation disappeared, a red cue box (6.6° each side) appeared for 100 ms at either the left or right box position of the fixated location. This time exposure is too fast for the fish to react to the presence of the cue. After a variable SOA (200 ms, 700 ms or 1,300 ms), a red target asterisk (3.3°) appeared for 3,000 ms or until a response was detected. The target could appear at the cued location (that is, same box location as the cue) or at the opposite location (that is, fixation location but not the same box as the cued box). After the target disappeared, a blank screen interval was presented between trials for 10 s. After the training period, we run each fish on the task for a period of about 2 months. Sessions in which the fish responded on <14 trials were excluded from the analyses. Each fish preformed 14 complete sessions. On some of the trials the fish did not respond. The amount of trials in which each fish responded was 230, 274 and 249 (for fish 1, 2 and 3, respectively). In every session, average RT was computed for the correct trials for every experimental condition. Behavioural experiments with humans Ten volunteers, all students at Ben-Gurion University of the Negev, participated in the experiment. The procedure was identical to that of the first experiment except for the following differences: (1) Every participant preformed 96 experimental trials. (2) The duration between trials was shortened to 1,000 ms. (3) Participants responded to the target appearance by pressing a keyboard key according to the target location (Q for left and P for right). (4) Participants preformed 8 practice trials before the experimental block. Trials in which participants responded incorrectly were excluded from the analyses (<2%). Since no fixation restrictions were employed for the fish, the human participants were not instructed to maintain fixation. How to cite this article: Gabay, S. et al. Inhibition of return in the archer fish. Nat. Commun. 4:1657 doi: 10.1038/ncomms2644 (2013).